Glycosylortho-(1-phenylvinyl)benzoates versatile glycosyl donors for highly efficient synthesis of bothO-glycosides and nucleosides Both of O -glycosides and nucleosides are important biomolecules with crucial rules in numerous biological processes. Chemical synthesis is an efficient and scalable method to produce well-defined and pure carbohydrate-containing molecules for deciphering their functions and developing therapeutic agents. However, the development of glycosylation methods for efficient synthesis of both O -glycosides and nucleosides is one of the long-standing challenges in chemistry. Here, we report a highly efficient and versatile glycosylation method for efficient synthesis of both O -glycosides and nucleosides, which uses glycosyl ortho -(1-phenylvinyl)benzoates as donors. This glycosylation protocol enjoys the various features, including readily prepared and stable donors, cheap and readily available promoters, mild reaction conditions, good to excellent yields, and broad substrate scopes. In particular, the applications of the current glycosylation protocol are demonstrated by one-pot synthesis of several bioactive oligosaccharides and highly efficient synthesis of nucleosides drugs capecitabine, galocitabine and doxifluridine. Carbohydrates are essential molecules with important rules in numerous biological processes such as cell growth and proliferation, immune response, and viral and bacterial infection [1] , [2] . Due to the highly heterogeneous character of carbohydrate structures, it is a formidable task to isolate homogeneous and pure glycans from nature. Chemical synthesis is an efficient, reliable, and scalable means to produce well-defined glycans for deciphering their functions and developing pharmaceuticals [3] , [4] , [5] , [6] , [7] . During the past century, a variety of glycosylation methods have been developed to streamline the chemical synthesis of glycans [8] , [9] , [10] , [11] , [12] , [13] , [14] , [15] , [16] , [17] . In comparison with synthesis of O -glycosides, methods capable of efficient synthesis of nucleosides ( N -glycosides) are relatively limited. Nucleosides are also important molecules, which played such crucial roles in many cellular processes as enzyme metabolism and regulation, cell signaling, and DNA and RNA synthesis [18] . Nucleosides natural products and nucleosides analogs usually demonstrate potent anticancer, antiviral, and antibacterial activities [19] . The development of the efficient methods for the synthesis of nucleosides still remains a high priority to develop therapeutic agents such as anticancer and antiviral drugs, to explore DNA sequencing technique, and to understand their mechanisms of action [20] , [21] , [22] . Most of common O -glycosylation donors including glycosyl trichloroacetimidates [23] , trifluoroacetimidates [24] , chlorides/bromides [25] , phosphites [26] , thioglycosides [27] , sulfoxides [28] , sugar 1,2-anhydrides [29] , and n -pentenyl glycosides [30] have the only limited success for nucleosides synthesis (Fig. 1a ). The problems inherent to nucleosides synthesis mainly include the poor solubility and nucleophilicity of nucleobases, which results in the unfavorable competition for glycosylation with other nucleophilic species derived from the leaving group and promoters in the coupling reaction. Therefore, the development of glycosylation methods for highly efficient synthesis of both O -glycosides and nucleosides is highly desirable and one of the long-standing challenges in chemistry. Fig. 1: Glycosyl donors for synthesis of O -glycosides and nucleosides. Prior art and current glycosylation protocol. Highlighted in blue are leaving groups and nucleophilic acceptors and in red are glycosidic linkages cleaved and formed. Bn benzyl, Bz benzoyl, NIS N -iodosuccinimide, TMSOTf trimethylsilyl trifluoromethanesulfonate, MW microwave. Full size image A Vorbrüggen type reaction [31] , [32] , [33] is a famous method for the synthesis of nucleosides, which involves the glycosylation of sugar acetates with trimethylsilylated nucleobases under strong Lewis acid activation (Fig. 1b ). However, due to the stoichiometric use of strong Lewis acids, e.g. trimethylsilyl triflate and SnCl 4 , the limitations of this method are obvious, including: (1) the poor functional group compatibility of the strong Lewis acid; (2) the low coupling yields and moderate N9/N7 regioselectivity when purines are used; and (3) the issues of work-up and disposal, especially on preparative scale. To overcome these issues, Jamison’s group [34] introduced pyridinium triflate salts as efficient bronsted acid catalysts for nucleosides and nucleosides analogs synthesis (Fig. 1b ). Despite the success in nucleosides synthesis, sugar acetates are relatively poor donors for synthesis of O -glycosides. In 2008, Yu’s group [35] introduced a glycosylation method with glycosyl ortho -alkynylbenzoates (ABz) as donors and gold(I) complexes as catalysts. This Yu glycosylation enjoys mild glycosylation reaction conditions and has been successfully demonstrated in the total synthesis for complex O -glycosides natural products and nucleosides antibiotics [10] , [36] (Fig. 1c ). In 2019, the group of Yu [37] reported another highly effective and versatile glycosylation method with 3,5-dimethyl-4-(2′-phenylethynylphenyl)phenyl (EPP) glycosides as donors, which is suitable for efficient synthesis both of O -glycosides and nucleosides (Fig. 1d ). Notwithstanding these breakthroughs, the challenges still remain in this realm. For example, methods using readily prepared and stable glycosyl donors, cheap and readily available promoters, and mild reaction conditions are still limited. The number of leaving groups that could be combined to achieve multi-steps one-pot synthesiss of oligosaccharides is still rare [13] , [14] , [38] , [39] . Furthermore, general glycosylation methods suitable for industrial appllications with lower costs for efficient synthesis of both O -glycosides and nucleosides remain extremely rare. Herein, we report a highly efficient and versatile glycosylation method with glycosyl ortho-(1-phenylvinyl)benzoates (PVB) as donors for efficient synthesis of both O -glycosides and nucleosides (Fig. 1e ). Readily prepared and stable donors, cheap and readily available promoters, mild reaction conditions, good to excellent yields, and broad substrate scopes are highlighted in this glycosylation protocol. Furthermore, the applications of the current glycosylation protocol have been successfully demonstrated in the one-pot synthesis of several bioactive oligosaccharides and highly efficient synthesis of nucleosides drugs capecitabine, galocitabine, and doxifluridine (Fig. 1f ). Conditions optimization We commenced with the preparation of glycosyl PVB donors, which were readily prepared by condensation of sugar hemiacetals with the ortho -(1-phenylvinyl)benzoic acid in the presence of EDCI, DMAP, and i Pr 2 EtN ( Supplementary Methods ). It was noteworthy that the ortho -(1-phenylvinyl)benzoic acid was easily obtained by one-step Wittig methenylation of the cheap 2-benzoylbenzoic acid (0.1$/g) in excellent yield [40] . The resultant glycosyl PVB donors ( 1a–t ) are stable and stay inert on shelf for at least one month. 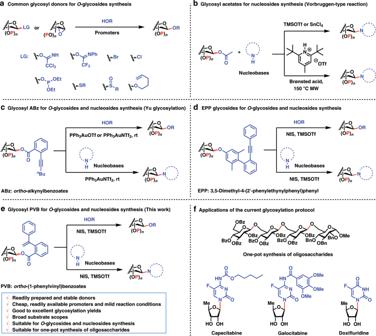Fig. 1: Glycosyl donors for synthesis ofO-glycosides and nucleosides. Prior art and current glycosylation protocol. Highlighted in blue are leaving groups and nucleophilic acceptors and in red are glycosidic linkages cleaved and formed. Bn benzyl, Bz benzoyl, NISN-iodosuccinimide, TMSOTf trimethylsilyl trifluoromethanesulfonate, MW microwave. Next, we investigated glycosylation of glucosyl perbenzoyl PVB 1a and 1,2:3,4-di- O -isopropylidene-α-galactoside 2a under various conditions (Table 1 ). A variety of promoters such as Ph 3 PAuOTf, AgOTf, Cu(OTf) 2 , TMSOTf and HOTf, and MeOTf were screened; however, glucosyl perbenzoyl PVB 1a stayed largely intact and no glycosylation reaction occurred, except the promoter HOTf affording the desired glycoside 3a in 9% yield. Fortunately, glycosylation of disarmed PVB 1a (1.2 equiv.) and galactoside 2a (1.0 equiv.) under the action of NIS (2.5 equiv.) and TMSOTf (0.3 equiv.) proceeded smoothly in CH 2 Cl 2 at 0 °C to RT, providing the coupled (1 → 6)-disaccharide 3a in 97% yield. Reducing the amount of NIS from 2.5 equiv. to 1.5 equiv. still produced disaccharide 3a in an excellent yiled (94%). The departing species, isobenzofuran-1-one derivative 4 was readily isolated and confirmed unambiguously by X-ray diffraction analysis (CCDC 1939909) (Fig. 2 ). Table 1 Conditions optimization for glycosylation with perbenzoyl glucosyl PVB 1a . Full size table Fig. 2: Scope of synthesis of O -glycosides with glycosyl PVB donors. Highlighted in blue are leaving groups and nucleophilic acceptors and in red are chemical bonds cleaved and formed. Ac acetyl, TIPS triisopropylsilyl, MP 4-methoxyphenyl, Cbz benzyloxycarbonyl, MS molecular sieves, RT room temperature. Full size image Scope of synthesis of O -glycosides With the optimal conditions for the model glycosylation reaction ( 1a + 2a → 3a ) in hand, we began to investigate the scope of this glycosylation protocol for O -glycosides synthesis (Fig. 2 ). We were pleased to discover that a wide range of carbohydrate alcoholic acceptors including the sterically hindered C4 position of glucose and C2 position of mannose were coupled smoothly with 1a , providing β-(1 → 6)-, (1 → 4)-, (1 → 3)-, and (1 → 2)-disaccharides 3b – h in excellent yields (92–99%). It is worth noting that this glycosylation protocol works well for both of higher and lower nucleophilic carbohydrate alcoholic acceptors (e.g., 3c and 3d ). A mild anesthetic menthol and hindered nucleophiles such as 1-adamantanol and benzyl oleanolate were also glycosylated uneventfully with 1a , producing the coupled glycosides 3i–k in 87–95% yields. Glycosylation of the acid and base-sensitive and electron-rich podophyllotoxin [41] with 1a also proceeded smoothly to furnish the desired podophyllotoxin 4- O -glucoside 3l in 94% yield, which is the analog of the first-line antitumoral drugs etoposide and teniposide [42] , [43] . Furthermore, we investigated different glycosyl donors. For pyranosyl donors, a wide array of glycosyl PVB donors including d -galacto-, d -manno-, l -rhamno-, l -arabino-, l -fuco-, and d -xylopyranosyl donors were coupled successfully to provide the corresponding glycosides 3m–r in excellent yields (88–99%). Besides pyranosyl donors, furanosyl PVB donors including l -arabino-, d -ribo-, d -galacto-, and even d -fructofuranosyl donors were also glycosylated efficiently to furnish the corresponding glycosides 3s–3v in nearly quantitative yields. It was noted that the famous Schmidt glycosylation method [44] using trichloroacetimidate (TCAI) as donors was not suitable for fructosylation due to the unsuccessful preparation of fructosyl trichloroacetimidate under various basic conditions [45] . The peracetyl gluco-, rhamno-, and xylopyranosyl PVB donors ( 1b , 1f and 1h ) reacted uneventfully with secondary and primary sugar alcohols to give the corresponding glycosides 3w–3y in 96–99% yield. It is noteworthy that when the corresponding glucosyl ABz was used as a donor, the complex mixture was obtained due to the production of orthoester-derived byproducts [46] . For both superarmed and armed glycosyl PVB donors [47] , while 3z–3ab were produced as the only β-products in 87–99% yields, an anomeric mixture of the glycoside 3ac was isolated expectedly (99%, α / β = 1:1). For the formation of the challenging 2-deoxy glycosidic linkages, glycosyl PVB donor 1s was also a viable substrate, and 3ad was produced efficiently in 86% yield. N-glycosylation of pyrimidine nucleobases After the glycosyl PVB glycosylation protocol for efficient synthesis of O -glycosides was successfully set up, the N-glycosylation of pyrimidine nucleobases with glycosyl PVB was then investigated (Fig. 3 ). Treatment of the poorly soluble uridine 5a (2.0 equiv.) with N , O -bis(trimethylsilyl)trifluoroacetamide (BSTFA) in acetonitrile produced the soluble silylated uridine. We found that it was necessary to heat the nucleobases to 50 °C in 30 min to insure the full solubility of nucleobases. The resulting soluble silylated uridine was coupled with the perbenzoyl ribofuranosyl PVB 1l in the activation of NIS (1.5 equiv.) and TMSOTf (0.5 equiv.) at 0 °C to room temperature. To our good fortune, the reaction proceeded smoothly, providing the desired nucleoside 6a cleanly in an excellent yield (93%). With the optimal condition for the N-glycosylation of pyrimidine nucleobases in hand, we began to investigate the scope of this glycosylation protocol. We were pleased to discover that a wide range of nucleobases including uridine 5a , thymine 5b , N 4-benzoylcytosine 5c , 5-fluorouridine 5d , and trifluorothymine 5e were glycosylated smoothly with ribofuranosyl donors 1l and 1t , affording the desired nucleosides 6a–e in excellent yields (85–96%). In comparison, using Yu glycosylation with glycosyl ABz, nucleosides 6a , 6b , and 6c were obtained in 85%, 88%, and 95% yields, respectively [36] . Using EPP glycosides, 6a and 6c were produced in 90% and 91% yields, respectively [37] . The other furanosyl donors 1k and 1m–n including l -arabino, d -galacto-, and even d -fructofuranosyl donors were also coupled efficiently with nucleobases 5a , 5c , and 5e , providing the corresponding nucleosides 6f–h in excellent yields (91–96%). Besides the furanosyl donors, the pyranosyl PVB donors 1a , 1e , 1g , and 1i including d -gluco-, l -rhamno-, l -arabino-, and d -xylopyranosyl donors were also glycosylated smoothly with 5-fluorouridine 5d and trifluorothymine 5e , furnishing the corresponding nucleosides 6i–n in excellent yields (89–99%). Interestingly, the big value (9.4 Hz) of the J 1,2 of nucleoside 6j suggests a α- l -rhamnopyranose in 4 C 1 conformation with the diaxial orientation of H 1 and H 2 . It is noted that the fluoro and trifluoromethyl groups are intriguing structural motifs and frequently found in many pharmaceuticals. Thus, the incorporation of fluoro and trifluoromethyl groups into nucleosides may have great potential for the development of therapeutic agents [48] , [49] . Fig. 3: Scope of synthesis of nucleosides with glycosyl PVB donors. Highlighted in blue are leaving groups and nucleophilic acceptors and in red are glycosidic bonds cleaved and formed. Boc t -butoxycarbonyl. Full size image N-glycosylation of purines nucleobases We then examined the N-glycosylation of purines nucleobases with glycosyl PVB, which was a challenging task due to the N9/N7 regioselectivity issues of purines in the glycosylation reactions [50] , [51] . We chose two purine nucleobases, namely, N 6-bis( tert -butoxycarbonyl)adenine 5f and N 2- tert -butoxycarbonyl-2-amino-6-iodopurine 5g , which have already been efficiently utilized in Yu glycosylation of purines [36] and Mitsunobu-type N-alkylation reactions [52] with high N9/N7 regioselectivity. Tert -butoxycarbonyl (Boc) group installed in purines 5f and 5g solved the solubility issues of purine nucleobases and enabled the glycosylation to be conducted in dichloromethane. Boc-protected purine 5f (1.0 equiv.) was glycosylated with the perbenzoyl ribofuranosyl PVB 1l (1.2 equiv.) in the promotion of NIS (1.5 equiv.) and TMSOTf (0.3 equiv.) in dichloromethane at −20 °C. To our delight, the reaction proceeded efficiently, furnishing the desired N9 nucleoside 6o in an excellent yield (84%). Coupling of N 2-Boc-2-amino-6-iodopurine 5g with PVB 1l also led to the corresponding N9 6-iodopurine nucleoside 6p in 85% yield, which is a useful precursor to the corresponding guanine nucleosides or 6-substituted analogs [52] , [53] . With the optimal condition for N-glycosylation of purines in hand, we went on to investigate the scope of this glycosylation protocol (Fig. 3 ). We were delighted to find that a wide array of furanosyl donors, including l -arabino-, d -5-deoxyribo-, d -galacto-, and even d -fructofuranosyl donors, were coupled smoothly, providing the desired N9 nucleosides 6q–t in excellent yields (82–85%). Besides furanosyl donors, the pyranosyl donors including d -gluco-, d -galacto-, d -manno-, l -arabino-, d -xylo-, and l -rhamnopyranosyl donors also led to the coupled N9 nucleoside products 6u–z in satisfactory yields (66–76%). Interestingly, nucleoside product 6w bears a α- d -mannopyranose in 1 C 4 conformation [54] , [55] , [56] . It was noted that N-glycosylation of purines using Yu glycosylation with glycosyl ortho -alkynylbenzoates afforded N9 nucleosides 6o , 6p , 6q , and 6u in 77%, 84%, 80%, and 48% yield, respectively [36] . Using EPP glycosides, the corresponding 6o , 6q , and 6u were prepared in 74%, 73%, and 69% yields, respectively [37] . Comparison of the donor reactivities Of note, the present glycosyl PVB activation conditions (NIS/TMSOTf) have been extensively utilized in thioglycosides and 4- n -pentenyl glycosides glycosylation reactions [57] , [58] . Therefore, the donor reactivities of glycosyl PVB with thioglycosides and 4- n -pentenyl glycosides were compared (Fig. 4 ). NIS (1.0 equiv.) and TMSOTf (0.3 equiv.) were added to a mixture of p -tolylthio perbenzoyl glucopyranoside ( 7a , 1.0 equiv. ), perbenzoyl glucopyranosyl PVB ( 1a , 1.0 equiv. ), and sugar alcohol ( 2a , 1.0 equiv.) in CH 2 Cl 2 at −15 °C. Interestingly, after 2 h, p -tolylthio perbenzoyl glucopyranoside 7a was fully recovered (98%), while perbenzoyl glucopyranosyl PVB 1a was completely glycosylated with 2a , providing the coupled disaccharide 3a and isobenzofuran-1-one derivative 4 in 94% and 99% isolated yield, respectively. Furthermore, we compared the donor reactivity of disarmed PVB donor 1a with armed perbenzyl glucothioglycoside, which shows about 2000 times reactivity of its perbenzoyl counterpart 7a [59] . To our surprise, disarmed PVB donor 1a was still more reactive and about three times reactivity of perbenzyl glucothioglycoside 7b (Supplementary Fig. 7 ). 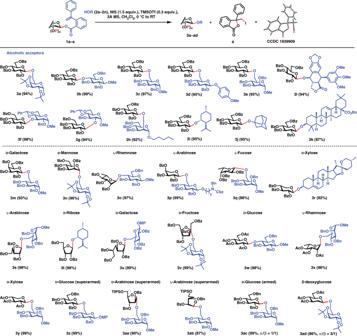Fig. 2: Scope of synthesis ofO-glycosides with glycosyl PVB donors. Highlighted in blue are leaving groups and nucleophilic acceptors and in red are chemical bonds cleaved and formed. Ac acetyl, TIPS triisopropylsilyl, MP 4-methoxyphenyl, Cbz benzyloxycarbonyl, MS molecular sieves, RT room temperature. In a similar competition reaction, while 1a was fully coupled with 2a , producing 3a and 4 in a nearly quantitatively yield, perbenzoyl glucosyl n -Pen 7c was recovered completely (99%). Furthermore, 1a was about seven times more reactive than perbenzyl glucosyl n -Pen 7d (Supplementary Fig. 9 ). Fig. 4: Comparison of the donor reactivities and one-pot synthesis of oligosaccharides 13–16 . Highlighted in red, blue, and green are the corresponding leaving groups, activation conditions, and glycosidic bonds formed. Tol p -tolyl, ABz ortho -alkynylbenzoates, PVB ortho -(1-phenylvinyl)benzoates, Pen pentenyl, TCAI trichloroacetimidates. Full size image One-pot synthesis of oligosaccharides 13–16 We envisioned that large enough donor reactivity differences of glycosyl PVB donors with thioglycosides and 4- n -pentenyl glycosides could lead to one-pot synthesis of oligosaccharides. Indeed, for glycosyl PVB and thioglycoside pair, glycosylation of disarmed PVB donor 1a (1.0 equiv.) with disarmed thioglycoside 8 (1.0 equiv.) under the activation of NIS (1.0 equiv. ), and TMSOTf (0.3 equiv.) produced the coupled disaccharide intermediate, which was further coupled with the acceptor 2e (1.0 equiv.) under the promotion of NIS (1.5 equiv.) and TMSOTf (0.3 equiv. ), providing the trisaccharide 13 in 89% yield in the same pot (Fig. 4 ). For glycosyl PVB and n -Pen glycoside pair, PVB 1a (1.0 equiv.) was coupled with n -Pen 9 (1.2 equiv.) 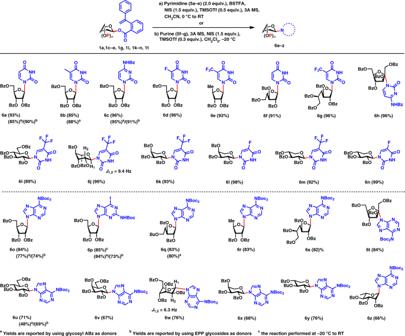Fig. 3: Scope of synthesis of nucleosides with glycosyl PVB donors. Highlighted in blue are leaving groups and nucleophilic acceptors and in red are glycosidic bonds cleaved and formed. Boct-butoxycarbonyl. under the promotion of NIS and TMSOTf to generate the coupled disaccharide intermediate, which was further glycosylated with the acceptor 2c (1.1 equiv.) under the action of NIS and TMSOTf, providing trisaccharide 14 in 73% yield in a one-pot manner. Orthogonal one-pot synthesis of oligosaccharides is one of the most popular one-pot glycosylation strategies [13] , [14] . However, the number of leaving groups that could be utilized in multistep orthogonal one-pot synthesis is still limited. Recently, the group of Xiao [38] developed orthogonal one-pot synthesis of oligosaccharides based on glycosyl ABz, which solved the shortcomings including aglycon transfer, high electrophilic character of departing species, and unpleasant odor inherent to thioglycosides based orthogonal one-pot glycosylation. We envisioned that orthogonal one-pot synthesis of oligosaccharides based on glycosyl PVB could also be explored to streamline chemical synthesis of oligosaccharides. Indeed, for glycosyl TCAI, ABz, and PVB triple, coupling of glucosyl TCAI 10 (1.2 equiv.) with ABz 11 (1.1 equiv.) under the catalysis of TMSOTf afforded disaccharide intermediate, which was further glycosylated with PVB 12 (1.0 equiv.) under the catalytic amount of Ph 3 PAuOTf, providing the trisaccharide intermediate. The above trisaccharide intermediate was further glycosylated with the acceptor 2c (0.9 equiv.) under the promotion of NIS and TMSOTf to give tetrasaccharide 15 in 74% yield in one-pot, whose sulfated derivatives exhibit significant proangiogenic activity [60] . It was noted that stepwise orthogonal glycosylation approach afforded tetrasaccharide 15 in only 39% overall yield [61] . 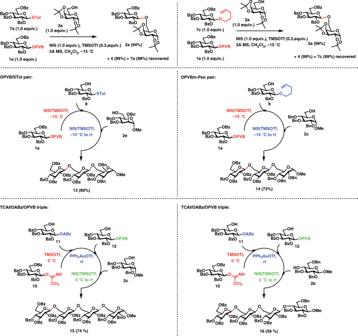Fig. 4: Comparison of the donor reactivities and one-pot synthesis of oligosaccharides13–16. Highlighted in red, blue, and green are the corresponding leaving groups, activation conditions, and glycosidic bonds formed. Tolp-tolyl, ABzortho-alkynylbenzoates, PVBortho-(1-phenylvinyl)benzoates, Pen pentenyl, TCAI trichloroacetimidates. Replacing the above acceptor 2c with the poor 4-OH acceptor 2b , tetrasacchaide 16 was still obtained in satisfactory 59% overall yield in one pot by successive coupling of TACI 10 , ABz 11 , PVB 12 , and acceptor 2b (Fig. 4 ). Synthesis of nucleosides drugs Finally, the utilities of this glycosylation protocol have been successfully demonstrated in the application to the efficient synthesis of nucleoside antibiotics capectibine, galocitabine, and doxifluridine (Fig. 5 ). In particular, capecitabine 17 is an important drug against breast and colorectal cancers [62] , [63] , [64] , [65] and is commercially available in the market under the brand name XELODA ® . Using the above standard conditions for N-glycosylation with pyrimidines, pyrimidine 5h was coupled efficiently with perbenzoyl 5-deoxyribofuranosyl PVB 1t , providing the pyrimidine nucleoside in excellent yield (91%), which was treated with NaOH in MeOH/H 2 O to produce nucleoside capecitabine 17 in 96% yield. It was noted that N-glycosylation of sugar acetate with pyrimidine 7 h under the action of pyridinium triflate salts at 140 °C developed by the group of Jamison [34] resulted in significant decomposition of carbamate functionality and moderate glycosylation yield [66] . This problem rendered them to first couple more electron rich and less reactive pyrimidine, then install the carbamate functionality, finally deprotect the acyl groups to achieve the synthesis of capectitabine 17 in 72% overall yield over three steps [66] . In comparsion, the current two-step synthesis of anticancer drug capecitabine 17 in 87% overall yield is clearly more efficient and less steps than any other previously reported processes [67] , [68] , [69] , [70] , [71] , [72] , [73] . The current glycosylation protocol highlighted the mild reaction condition, which is compatible with the carbamate functionality. In the similar glycosylation protocol, coupling of pyrimidines 5d and 5i with PVB 1t afforded the corresponding pyrimidine nucleosides in excellent yields (83–98%), which was deprotected with NaOH in MeOH/H 2 O to give doxifluridine 18 and galocitabine 19 in 91% and 95% yields, respectively. Fig. 5: Application to the synthesis of nucleosides Capecitabine 17, Doxifluridine 18, and Galocitabine 19. Highlighted in blue are leaving groups and nucleophilic acceptors and in red are glycosidic bonds formed. Full size image A plausible mechanism After the glycosyl PVB glycosylation protocols for highly efficient synthesis both of O -glycosides and nucleosides were successfully established and the synthetic applications toward one-pot synthesis of bioactive oligosaccharides and efficient synthesis of nucleosides antibiotics were successfully demonstrated, a plausible mechanism of the NIS/TMSOTf mediated glycosylation with glycosyl PVB as donors was outlined in Fig. 6 . Activation of NIS with TMSOTf leads to the formation of iodonium species, which can attack a C–C double bond within the aglycone of glycosyl PVB 1 , resulting in the generation of diphenylmethyl cation species A . We envisioned that this cation species A can be stabilized by two adjacent phenyl groups, facilitating the ready cleavage of the anomeric C–O bond to generate the glycosyl oxocarbenium species B and the departing species of the leaving group, isobenzofuran-1-one derivative 4 . The oxocarbenium B can be attacked by alcoholic nucleophiles 2 or nucleobases 5 to produce O -glycosides products 3 or nucleosides 6 and H + . Protonation of silylated succinimide regenerates TMSOTf, which can undergo the next catalytic cycle. Fig. 6: A plausible mechanism of the glycosyl PVB glycosylation protocol. Highlighted in red are active species and chemical bonds cleaved and formed; highlighted in blue are leaving groups and nucleophilic acceptors and in light blue are oxocarbenium intermediates. Full size image We have developed a highly efficient and versatile glycosylation method for the highly efficient synthesis of both O -glycosides and nucleosides, which uses glycosyl PVB as donors and NIS/TMSOTf as promoters. 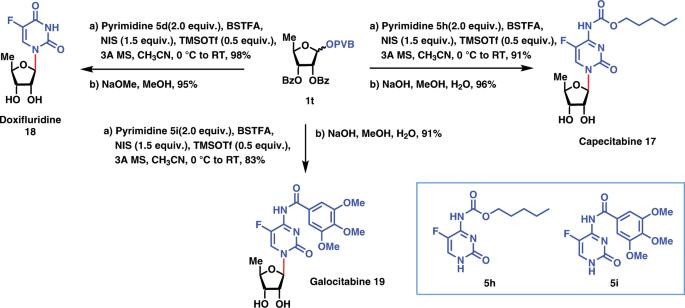Fig. 5: Application to the synthesis of nucleosides Capecitabine 17, Doxifluridine 18, and Galocitabine 19. Highlighted in blue are leaving groups and nucleophilic acceptors and in red are glycosidic bonds formed. 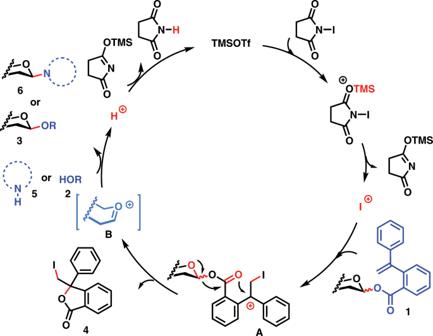Fig. 6: A plausible mechanism of the glycosyl PVB glycosylation protocol. Highlighted in red are active species and chemical bonds cleaved and formed; highlighted in blue are leaving groups and nucleophilic acceptors and in light blue are oxocarbenium intermediates. This glycosylation protocol highlighted the various advantages, including (1) readily prepared and stable glycosyl PVB donors; (2) cheap and readily available promoters, and mild reaction conditions; (3) good to excellent glycosylation yields; and (4) broad substrate scopes. Furthermore, one-pot synthesis of oligosaccharides based on glycosyl PVB highly streamlined chemical synthesis of oligosaccharides, which avoided three major issues including aglycon transfer, undesired interference of departing species, and unpleasant odor inherent to thioglycosides based one-pot glycosylation. Highly efficient synthesis of nucleosides drugs capecitabine, galocitabine, and doxifluridine using the current glycosylaton protocol has also been successfully demonstrated. With these exciting features, we believe this glycosylation protocol will find broad applications in chemical synthesis and inspire the development of other glycosylation methods for efficient synthesis of both O -glycosides and nucleosides. General The complete experimental details, compound characterization data, and NMR spectra of compounds synthesized in this study see Supplementary information. General procedure for glycosylation with alcoholic acceptors A solution of glycosyl PVB donor 1 (1.2 equiv.) and alcoholic acceptors 2 (1.0 equiv.) in dry CH 2 Cl 2 (0.033 M) was stirred at room temperature for 30 min in the presence of activated 3 Å MS (3.0 g/mmol) under argon atmosphere. Then the vessel was chilled to 0 °C, to which NIS (1.5 equiv.) and TMSOTf (0.3 equiv.) were added. The reaction mixture was stirred for 2 h after the temperature gradually rose to room temperature. Then Et 3 N was added to quench the reaction and the solvent was removed under reduced pressure. The resulting residue was purified by silica gel column chromatography to afford the glycosylated product. General procedure for glycosylation with pyrimidines BSTFA (4.0 eq) was added to a stirred suspension of pyrimidine acceptors 5a–e and 5h–i (2.0 equiv.) in dry CH 3 CN (0.1 M) under argon atmosphere. After the mixture was stirred at 50 °C for 30 min, this solution was added to a solution of glycosyl PVB donor 1 (1.0 eq) and activated 3 Å MS (4.0 g/mmol) in dry CH 3 CN (0.05 M), which has been stirred at room temperature for 30 min under argon atmosphere. The stirring was continued for 10 min, then the vessel was chilled to 0 °C, to which NIS (1.5 equiv.) and TMSOTf (0.5 equiv.) were added. The reaction mixture was stirred for 3 h after the temperature gradually rose to room temperature. Et 3 N was added to quench the reaction and the solvent was removed under reduced pressure. The resulting residue was purified by silica gel column chromatography to afford the glycosylated product. General procedure for glycosylation with purines A solution of glycosyl PVB donor 1 (1.2 equiv.) and purines acceptors 5f–g (1.0 equiv.) in dry CH 2 Cl 2 (0.033 M) was stirred at room temperature for 30 min in the presence of activated 3 Å MS (3.0 g/mmol) under argon atmosphere. Then the vessel was chilled to −20 °C, to which NIS (1.5 equiv.) and TMSOTf (0.3 equiv.) were added. The reaction mixture was stirred for 2 h after the temperature gradually rose to room temperature. Then Et 3 N was added to quench the reaction and the solvent was removed under reduced pressure. The resulting residue was purified by silica gel column chromatography to afford the glycosylated product.